Excitons versus free charges in organo-lead tri-halide perovskites Excitonic solar cells, within which bound electron-hole pairs have a central role in energy harvesting, have represented a hot field of research over the last two decades due to the compelling prospect of low-cost solar energy. However, in such cells, exciton dissociation and charge collection occur with significant losses in energy, essentially due to poor charge screening. Organic–inorganic perovskites show promise for overcoming such limitations. Here, we use optical spectroscopy to estimate the exciton binding energy in the mixed-halide crystal to be in the range of 50 meV. We show that such a value is consistent with almost full ionization of the exciton population under photovoltaic cell operating conditions. However, increasing the total photoexcitation density, excitonic species become dominant, widening the perspective of this material for a host of optoelectronic applications. Perovskite solar cells were first introduced in a dye-sensitized configuration, where the dye was replaced by organo-lead halide perovskite crystals (e.g. CH 3 NH 3 PbI 3 or CH 3 NH 3 PbI 3−x Cl x ) sensitizing the surface of mesoporous TiO 2 (refs 1 , 2 , 3 , 4 , 5 ). In the perovskite-sensitized configuration, developed within the excitonic solar cell concept, there is no requirement for long-range exciton or charge diffusion, as the perovskite crystals are sandwiched within a nanoscale heterojunction between an electron-accepting metal oxide (TiO 2 ) and a hole-accepting organic hole-transporter (or redox active electrolyte) and long-range transport occurs in those phases. Although the rapid advancement of this sensitized approach has occurred, there has been in parallel a striking divergence in technology, where the mesoporous TiO 2 has been proven non-essential [5] , and simply a solid absorber layer sandwiched within a planar heterojunction has been demonstrated to operate extremely well, with power-conversion efficiencies of over 15% already reported [6] , [7] . The perovskite absorbers thus appear capable of operating in a similar manner to excitonic absorbers, but also in a comparable configuration and with comparable performance to the best inorganic thin-film semiconductors [6] , [8] . The fundamental question that arises from these studies concerns the nature of the elementary photoexcitations that are involved in the photovoltaic (PV) mechanisms; in particular whether bound excitons are created and transport energy to the heterojunction, thus requiring further ionization at the heterojunction, or whether free charges are spontaneously generated within the bulk of the perovskite [9] , [10] , [11] , [12] . In order to answer this question, we explicitly need to know the exciton binding energy in the room temperature (RT) crystal phase of the perovskite absorber, and to understand the branching ratio between free carriers and excitons under operating solar cell conditions. In this work, we use the temperature dependence of the absorption band edge to estimate the exciton binding energy in CH 3 NH 3 PbI 3−x Cl x perovskite crystals. Subsequently, we use this value in the Saha equation, which governs ionization processes [13] , [14] , to estimate the equilibrium branching ratio between free charges and bound excitons as a function of temperature and charge density. We find that at equilibrium, following photoexcitation, there is a predominant fraction, near unity, of free charges in the PV operating regime. Temperature dependence of optical absorption In Fig. 1 , we show the optical absorption spectra taken in a broad temperature ( T ) range from RT=290 K to 4.2 K, on a polycrystalline film of CH 3 NH 3 PbI 3 and of its mixed-halide analogue CH 3 NH 3 PbI 3− x Cl x . We study both flat films deposited on glass, which are polycrystalline with crystal sizes larger than 500 nm in diameter [7] ( Fig. 1a,b ), and perovskite films infiltrated into a mesoporous oxide scaffold, where the perovskite crystals are on the order of 60 to 100 nm in size [7] ( Fig. 1c,d ). 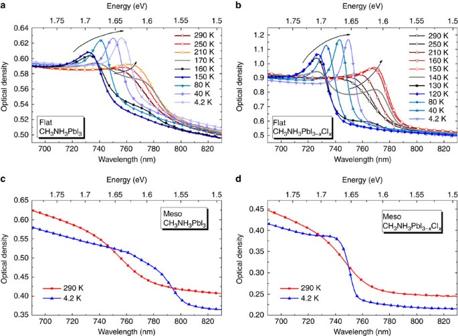Figure 1: Temperature dependence of the absorption spectra of the mixed-halide perovskites. Absorption spectra of CH3NH3PbI3and CH3NH3PbI3-xClxas a function of temperature (290–4.2 K). (a,b) Thin films on a glass substrate and (c,d) on a mesoporous Al2O3substrate. Figure 1a shows the spectra of the CH 3 NH 3 PbI 3 in a spectral range between 690 nm and 825 nm. A sharp peak at ~765 nm emerges at lower temperatures, which we attribute to an excitonic transition. At 170K, a second excitonic peak emerges at 740 nm. Upon further reduction of temperature, the latter peak gains strength in intensity and monotonically shifts to longer wavelengths, whereas the first peak disappears. We assign this behaviour to a phase transition of the perovskite crystal, notably from a tetragonal to an orthorhombic structure [15] , [16] , which commences at 170 K, inducing a blue shift in the absorption edge of about 60 meV, and completes at 150 K. Within this temperature range, the two phases coexist, possibly due to the polycrystalline nature of the sample. At 4.2 K a single excitonic feature peaks at~760 nm, similar to what has been observed in single crystals of CH 3 NH 3 PbI 3 (refs 17 , 18 ). Figure 1: Temperature dependence of the absorption spectra of the mixed-halide perovskites. Absorption spectra of CH 3 NH 3 PbI 3 and CH 3 NH 3 PbI 3- x Cl x as a function of temperature (290–4.2 K). ( a , b ) Thin films on a glass substrate and ( c , d ) on a mesoporous Al 2 O 3 substrate. Full size image At RT, however, we cannot observe a clear gap between the excitonic peak and the conduction band continuum. We also note that as the temperature increases, especially in the low-temperature stable crystalline phase, the absorption band edge blue shifts. This ‘Varshni’ trend is often observed in lead composite semiconductors with a positive thermal expansion coefficient of the band gap, d E g /d T [19] , [20] . The CH 3 NH 3 PbI 3− x Cl x perovskite absorption spectra are presented in Fig. 1b . They show a similar trend in temperature, with evident positive d E g /d T in the low-temperature phase; however, some important differences exist. First of all, the phase transition is activated at a lower temperature (~140 K), and is completed by 120 K, probably due to different chemical/structural environments in the two compounds. Secondly, the excitonic peak emerges with a stronger intensity with respect to the broad continuum (see spectrum at 4.2 K). A different scenario appears when looking at the absorption spectra of the perovskite crystallites formed in the mesoporous Al 2 O 3 scaffold ( Fig. 1c,d ), which imposes a smaller crystal size of the crystals [7] . Both materials show a broad band edge with no evident excitonic peak and are blue shifted with respect to the flat samples. The structural phase transition can still be observed at the same temperature for the CH 3 NH 3 PbI 3− x Cl x (see Supplementary Fig. 1 in the SI where the complete temperature range is reported). However, upon cooling, the spectra remain featureless. Thus, smaller crystals show virtually no resolvable excitonic transition. We can exclude any confinement phenomena as in this case one would expect an opposite trend, that is, appearance of the exciton optical transition as the crystal size is reduced. On the other hand, the reduction in size, the enhancement of the surface area and the presence of a scaffold during the crystallization process is likely to increase the relative contribution of surface effects, which may result in structural strains and/or doping mechanisms, which notably reduce the exciton binding energy [21] . Interestingly, when we fabricate a combination of the above sample structures, that is, a thin ~80 nm interpenetrated mesostructured composite covered by a ~350 nm flat perovskite capping layer (see cartoon in Fig. 2a ), as is the case for the optimized device presented in ref. 7 , the resulting absorption spectrum is a combination of the absorption spectra of the two layers ( Fig. 2b ). This suggests that the presence of the thin mesoporous interlayer is responsible for tuning the optoelectronic properties of the material by tuning the crystal size. This may have important consequences for device performance, where generally higher photovoltages are obtained for mesostructured devices than for planar structures [7] . 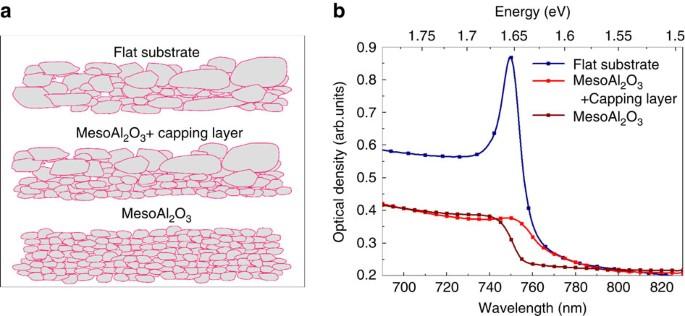Figure 2: Absorption spectra of mesostructured thin films. (a) Schematic presentation of the average crystals dimension for differently prepared samples, that is, deposited on a glass substrate (top), on a thick Al2O3scaffold without a perovskite capping layer (bottom) and a thin Al2O3scaffold with a perovskite capping layer (middle). (b) Absorption spectra of CH3NH3PbI3−xClx,thin films collected at 4.2 K. The films were deposited on a flat glass substrate (blue line), a thick mesoporous Al2O3(dark red line) and according to the optimized device structure where part of the perovskite film is infiltrated in the mesoporous Al2O3and an additional crystalline perovskite capping layer is present7(red line). For better comparison, spectra are offset. Figure 2: Absorption spectra of mesostructured thin films. ( a ) Schematic presentation of the average crystals dimension for differently prepared samples, that is, deposited on a glass substrate (top), on a thick Al 2 O 3 scaffold without a perovskite capping layer (bottom) and a thin Al 2 O 3 scaffold with a perovskite capping layer (middle). ( b ) Absorption spectra of CH 3 NH 3 PbI 3− x Cl x , thin films collected at 4.2 K. The films were deposited on a flat glass substrate (blue line), a thick mesoporous Al 2 O 3 (dark red line) and according to the optimized device structure where part of the perovskite film is infiltrated in the mesoporous Al 2 O 3 and an additional crystalline perovskite capping layer is present [7] (red line). For better comparison, spectra are offset. Full size image Exciton binding energy estimation The optical analysis presented above suggests the presence of an excitonic transition, probably very close to the continuum. Indeed, the presence of a Wannier–Mott exciton with a binding energy of about 45 meV has been predicted in the single crystal of CH 3 NH 3 PbI 3 at low temperatures [17] , [18] . Temperature-dependent, time-resolved photoluminescence (PL) is one approach for estimating the exciton binding energy in a semiconductor. We indeed observed a reduction in PL intensity of CH 3 NH 3 PbI 3− x Cl x when increasing the temperature; however, the PL dynamics did not allow for an unambiguous assignment to the enhancement in thermal dissociation rate of excitons at higher temperatures. As such, here, we estimate an upper limit of the exciton binding energy in CH 3 NH 3 PbI 3− x Cl x , by using the temperature-dependent absorption line width of the observed excitonic transition. As inhomogeneous broadening due to disorder is generally temperature independent, here we only take into account the homogeneous broadening mechanism within the two-level system [22] . The coherence lifetime T 2 of the excited state transition can be affected by the natural population decay of the excited state ( T 1 ) and by elastic scattering events (with rate γ) that do not change the excited state population but contribute to the broadening of the transition. For most polar inorganic solids at high temperatures (for example, T >100 K), phonon interaction leads predominantly to exciton ionization (through inelastic scattering) [22] , [23] . This approximation is valid in our case, as the exciton absorption broadening occurs together with a reduction in the intensity of the optical excitonic transition, thus the population decay rate, 1/ T 1, can be described as the sum of an intrinsic decay rate ( k 0 ) and thermal dissociation rate ( k T ) [22] , We model the rate of exciton thermal dissociation ( k T ) according to the following equation, where E B is the exciton binding energy, k B is the Boltzmann constant and ν T is the attempt frequency. Substituting the relationship between T 1 and T 2 , (ref. 22 ), into the equation for the line width, Δ ν =1/π T 2 we obtain: where Δ v 0 accounts for the temperature-independent broadening. For a better fit of the temperature dependence of the experimental line width h Δ v , the linear form of equation (3) is considered: In Fig. 3 , the natural logarithm of the excitonic transition line width of CH 3 NH 3 PbI 3− x Cl x is plotted as a function of the inverse of temperature in the range between 150 K and 290 K. The data are visualized in such a scale to emphasize the match between the experimental trend and the theoretical model. By fitting the data with equation (4), ( Fig. 3 ), we estimate an exciton binding energy of 55±20 meV. The fits are shown in Fig. 3 along with the experimental data. For statistical relevance, the points reported in the graph are derived from repeated measurements of many different samples. Details of the analysis are presented in section Supplementary Methods of the SI. 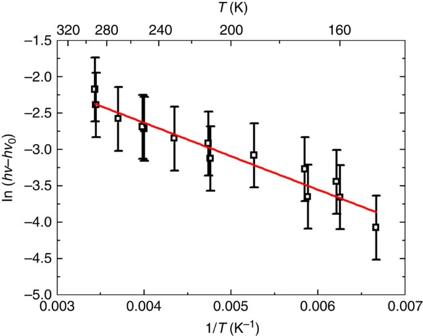Figure 3: Estimation of the exciton binding energy. Plot of the exciton absorption band broadeninghΔνin CH3NH3PbI3−xClxflat layer vs inverse temperature (150K<T<290K). For each point, the error bar indicates the maximum variation of the experimental value due to the ±10 K uncertainty in the determination of the sample temperature. The solid line is the fit realized according to equation (4), which gives an estimation for the binding energy ofEB=(55±20) meV and an attempt frequency of (7 fs)−1.χ2=0.92. Figure 3: Estimation of the exciton binding energy. Plot of the exciton absorption band broadening h Δ ν in CH 3 NH 3 PbI 3− x Cl x flat layer vs inverse temperature (150K<T<290K). For each point, the error bar indicates the maximum variation of the experimental value due to the ±10 K uncertainty in the determination of the sample temperature. The solid line is the fit realized according to equation (4), which gives an estimation for the binding energy of E B =(55±20) meV and an attempt frequency of (7 fs) −1 . χ 2 =0.92. Full size image Numerical simulation of the fraction of free charges vs excitons Under thermodynamic equilibrium, there is a coexistence of free charges and excitons, and an interchange between the two species. The fraction of free charges ( n FC ) vs. excitons ( n exc ) is not only determined by the binding energy, which determines how long electron-hole pairs remain bound, but also by the excitation density ( n ), which influences how often electrons and holes meet to form excitons [13] , [14] . In the PV working regime, the total excitation density can be estimated from the absorbed solar flux and the excitation lifetime. We can estimate the absorbed solar flux by integrating the absorption of the perovskite film over the 100 mWcm −2 AM1.5 solar spectrum. The species lifetime can be estimated by measuring the PL decay in neat perovskite films (equivalent to operation under open-circuit conditions with ideal n- and p-type contacts that introduce no additional non-radiative decay channels) or in perovskite films contacted by a selective hole- or electron acceptor (similar to the scenario in the operating solar cells), which we have measured to be~270 ns and 5 ns, respectively [24] . We hence determine the steady state excitation density (where excitations can be free charge or excitons) to be between 10 13 and 10 15 cm −3 . If we assume a dielectric constant of 6.5 (ref. 18) [18] and a binding energy of approximately 50 meV, the exciton radius can be calculated to be ~2.3 nm. Considering this value (in agreement with ref. 15 ) we can neglect exciton–exciton interaction, which only occurs for n >10 20 cm −3 , because there is essentially no wavefunction overlap. Consequently, we can safely assume that the binding energy is independent of excitation density [23] , [25] . Within such an approximation, we can apply the law of mass action for Wannier–Mott excitons, as described by the Saha–Langmuir equation [13] , [14] . The fraction of free charges over the total density of excitation, x , for a 3D semiconductor can be expressed as [13] : where E B is the exciton binding energy, μ is the reduced mass of the exciton (approximated to 0.15 m e (ref. 18 ), see Supplementary Fig. 2 for modelling as a function of reduced exciton mass), h is Planck’s constant, T is temperature and n is the total density of excitation, n = n FC + n exc . The form of this equation is quite intuitive; the higher the temperature, the greater the ratio of free charge to excitons, but the higher the density of excitations, the lower the ratio of free charge due to the greater possibility for free electron-hole capture events. In Fig. 4a , we model the fraction of free charges over a wide range of total photoexcitation densities. Our key finding is that at RT, at excitation densities that may be realistic for operating solar cells ( n <10 15 cm −3 ), free charges represent the dominant population. The model shows that upon temperature reduction, the exciton population starts to increase, becoming dominant below 120 K (see Fig. 4b ) [13] . 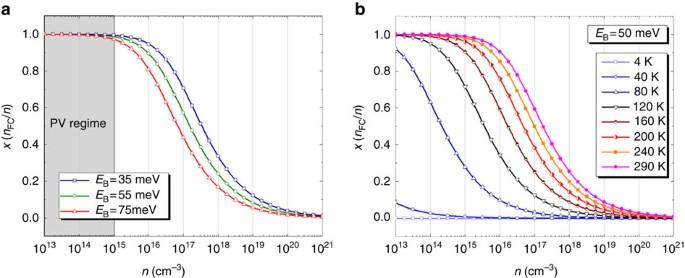Figure 4: Modelling of the fraction of free charges over the total photoexcitation. (a) Simulation of the free charge fraction over the total excitation density (x=nFC/n) at thermal equilibrium according to equation (5) described in the text. For this simulation, we used an exciton binding energy of (55±20) meV and an exciton reduced mass,μ=0.15me(ref.18). The shaded area represents PV operating conditions (PV regime). (b) Simultaion at different temperatures. With an exciton reduced massμ=0.15mefrom ref.18and the estimated binding energy of 50 meV. Figure 4: Modelling of the fraction of free charges over the total photoexcitation. ( a ) Simulation of the free charge fraction over the total excitation density ( x = n FC / n ) at thermal equilibrium according to equation (5) described in the text. For this simulation, we used an exciton binding energy of (55±20) meV and an exciton reduced mass, μ =0.15 m e (ref. 18 ). The shaded area represents PV operating conditions (PV regime). ( b ) Simultaion at different temperatures. With an exciton reduced mass μ =0.15 m e from ref. 18 and the estimated binding energy of 50 meV. Full size image We have identified that the exciton binding energy in the organo-lead mix-halide perovskite is 55±20 meV. This indicates that free charges are predominantly generated and are responsible for PV operation following light absorption, akin to a conventional inorganic semiconductor thin-film solar cell. This indicates that the role of the heterojunction in the perovskite solar cells is simply to enable selective charge collection, and not to facilitate exciton ionization. Notably, while perovskite cells are not excitonic in their operating principles, they still preserve a large absorption oscillator strength at the band edge, reminiscent of the underlying excitonic transition. This is a clear advantage in light harvesting near the band edge, enabling extremely thin-film solar cells to fully absorb light across the solar spectrum, and is in part responsible for the exceptional performance of the planar heterojunction perovskite solar cells [9] . Moreover, according to what we have shown, tuning the total density of photoexcitation allows for tuning of the nature of the primary photoexcitation at the thermodynamic equilibrium, that is, from free charges to excitons, thus opening up the way for application of these intriguing materials to a host of optoelectronic devices. Sample preparation Glass substrates were cleaned sequentially in 2% hallmanex detergent, acetone, propan-2-ol and oxygen plasma. The compact TiO 2 layer (~50 nm) was deposited by spin coating (at 2,000 r.p.m. for 60 s) a mildly acidic solution of titanium isopropoxide in ethanol, followed by annealing at 500 °C for 30 min. The ~0.5 μm TiO 2 and Al 2 O 3 mesoporous layers were deposited by spin coating from stock solutions followed by sintering at 550 °C for 30 min, as described previously [3] , with appropriate dilutions to give the thin mesoporous Al 2 O 3 layer (~80 nm). The perovskite precursor solutions were prepared using methods described previously for the mixed halide [3] . In brief, the CH 3 NH 3 PbI 3−x Cl x or CH 3 NH 3 PbI 3 precursor solutions were formed by dissolving methylammonium iodide and either lead (II) chloride (Sigma-Aldrich) or lead (II) iodide (Sigma-Aldrich) in anhydrous N , N -DimethylformamideDMF at a 3:1 molar ratio of MAI to PbCl 2 /PbI 2 , with final concentrations of 0.88 M lead chloride/iodide and 2.64 M methylammonium iodide. The perovskite layer was then formed by spin coating the precursor solutions directly on the glass substrate, compact layer or the mesoporous layer at 2,000 r.p.m. in air. The flat and thin meso samples were spin coated without dilution but mesoporous samples were spin coated from diluted (three parts in four) precursor solutions. After spin coating, the CH 3 NH 3 PbI 3−x Cl x films were annealed at 100 °C for 45 min, and the CH 3 NH 3 PbI 3 at 150 °C for 15 min. For the flat and thin mesoporous samples (that is, those without thick mesoporous layers), the perovskite films were sealed by spin coating a layer of the insulating polymer poly(methylmethacrylate)(10 mg ml −1 , 1,000 r.p.m. ; Sigma-Aldrich) on top in order to ensure air- and moisture-insensitivity. Ultraviolet–visible absorption Absorption measurements were performed using a spectrophotometer (Perkin Elmer Lambda 1050) and a continuous flow static exchange gas cryostat (Oxford Instruments Optistat CF). The cryostat consist of three chambers, one inside the other. The sample is housed inside the internal chamber filled with gaseous He. The cryogenic liquid (He) is fluxed inside the second chamber allowing temperature control of the He atmosphere of the sample chamber. Eventually, a third chamber is evacuated (~10 −5 –10 −6 mbar) in order to assure thermal isolation from the external ambient. How to cite this article: D’Innocenzo, V. et al . Excitons versus free charges in organo-lead tri-halide perovskites. Nat. Commun. 5:3586 doi: 10.1038/ncomms4586 (2014).